Phase-transition-driven growth of compound semiconductor crystals from ordered metastable nanorods In polycrystalline semiconductors, grain boundaries are often sites with prevalence for electron-hole recombination and various strategies have been followed to minimize grain boundary areas. Generally, large grains or epitaxial films can be obtained at high temperatures. However, high growth temperatures limit the choice of substrate materials and can prove elusive for semiconductors comprising volatile elements such as kesterite Cu 2 ZnSnS 4 . Here we show that this limitation can be overcome by a transition of a matrix of densely packed metastable nanorods into large stable grains. Real-time analysis reveals that the grain growth is driven by a direct, isocompositional solid-state phase transition. Following this route, semiconductor films with a large-grained microstructure can be achieved within a few seconds at relatively low temperatures. Grain size as well as electrical and optical properties of the resulting films can be controlled via the heating rate. This synthesis route opens new possibilities for the fabrication of semiconductor crystals for photoelectric devices with tailored microstructures. Rapid advances in the growing field of nanocrystal synthesis as well as self-organization of supercrystals consisting of nanocrystals [1] , [2] , [3] , [4] , [5] open new pathways for the fabrication of materials and devices with tuned nano- and microstructures [6] , [7] . Recently, it has been found that the size and shape of large silver crystals can be tailored by coalescence of ordered precursor nanoparticles [3] . The perspective to tailor semiconductor crystals in a similar way is attractive as it would open new possibilities for the fabrication of microstructured optoelectric devices and semiconductor films with controlled morphology. Among the large family of zinc-blende related semiconductor materials, the compound semiconductor Cu 2 ZnSnS 4 (CZTS) is of particular interest having a high absorption coefficient coupled with earth abundance of its constituent elements and tunability of its physical properties by alloying with related compounds [8] , [9] , [10] . Hence, CZTS has recently been intensely studied as a photovoltaic absorber material [8] , [11] , [12] , [13] . However, the growth of large grained, homogenous CZTS films with controlled composition has proven difficult [14] , [15] , [16] . A multitude of synthesis strategies have been investigated to tackle this problem. In many cases, long annealing times at high temperatures and pressures or the addition of supplemental elements to further assist grain growth via secondary phases or doping is required, thereby changing the composition and properties [13] , [17] . More recently, the generation of CZTS in size-controlled nanocrystal form has attracted increasing attention allowing for low energy and scalable processing with excellent composition control [18] , [19] , [20] . However, in contrast to the coalescence of silver nanocrystals, which occurs already at low temperatures of 50 °C (ref. 3 ), significant direct coalescence of sulphur-based compound semiconductor nanocrystals such as CZTS has not been observed even at high temperatures of 500 °C (refs 21 , 22 ). For these chalcopyrite and kesterite nanocrystals, partial conversion into large grains is achieved only after annealing in selenium vapour, accompanied by a diffusion limited anion-exchange reaction [23] , [24] , [25] . In this paper, we demonstrate that this limitation for the fabrication of polycrystalline compound semiconductors with controlled microstructure can be surpassed: a direct, isocompositional and complete transition from CZTS nanocrystals to large-grained CZTS films can be achieved within a few seconds at relatively low temperatures by annealing a template of highly ordered nanorods of the metastable wurtzite-type polymorph of CZTS. As the wurtzite phase is not stable in the bulk, it presents a low barrier for rapid conversion to the desired kesterite phase with complete composition control. We show by high-resolution real-time diffraction that the growth of kesterite grains is triggered by this phase transition. The key properties that enable fast phase transition and grain growth are: the close structural relation of the hexagonal wurtzite phase to the final kesterite structure; the similar density and equal composition, which minimizes diffusion during the reaction; and the fact that the orientation of stable kesterite surfaces are—despite these similarities—different from that of the wurtzite nanorods. As these prerequisites are fulfilled by all wurtzite polymorphs of the various zinc-blende derived structures—such as ZnS, ZnO, CdTe, Cu(In,Ga)Se 2 , Cu 2 ZnSnS 4 and its relatives—the presented model of phase-transition-driven grain growth can be expected to apply to a large number of technologically important semiconductor materials. Nanorod precursor films CZTS nanorods were synthesized by a hot-injection method adapted from our previous report [20] (see Methods for details). These nanorods show good monodispersity with a diameter of 9±0.5 nm and a length of 35±1 nm ( Fig. 1a ) as well as a highly crystalline structure with elongation in direction of the c-axis of a hexagonal lattice ( Fig. 1b ). The nanorods were deposited perpendicularly on Mo-coated glass by electrophoresis, during which they form a self-organized close-packed superlattice ( Fig. 1c ). A large number of such nanorod layers were deposited to obtain a 1 μm thick nanorod film ( Fig. 1d ). X-ray diffraction (XRD) confirms a hexagonal wurtzite structure ( Fig. 1e ) with space group P6 3 mc, which was already reported before [20] , [26] (see Supplementary Fig. 1a for a larger angle range). In the literature nanocrystals with orthorhombic wurtz-stannite and pseudo-orthorhombic wurtz-kesterite structures are reported [27] , [28] , [29] , [30] , [31] , which produce similar diffraction signals due to a similar hexagonal anion sublattice, but differ in the ordering of the cations [30] . In our measurements, additional reflexes that indicate presence of wurtz-stannite or wurtz-kesterite instead of hexagonal wurtzite structure are not observed. 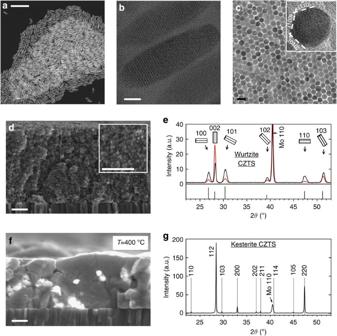Figure 1: CZTS nanorods and nanorod films before and after annealing. (a) Low resolution angular dark field transmission electron microscopy image (DFTEM) of nanorods (scale bar, 100 nm). (b) High-resolution transmission electron microscopy (HRTEM) image of a single rod (scale bar, 5 nm). (c) Top-down low resolution transmission microscopy (LRTEM) image of a monolayer sheet of vertically assembled nanorods. Inset: top-down view of a single nanorod by HRTEM (scale bar, 20 nm). The sidewalls of a nanorod are formed by lattice planes of the {100} family of the hexagonal lattice. (d) Cross-sectional scanning electron microscopy (SEM) image of a nanorod film (scale bar, 200 nm). (e) Diffractograms, measured by XRD under symmetric configuration, of two nanorod films with a high (red line) and a low (black line) degree of vertical alignment. Reference lines presenting random orientation are taken from Luet al.26The nanorod drawings indicate the orientation of the nanorods within the film that contribute to the corresponding reflexes. (f) SEM image of a cross-section of a nanorod film after annealing at 400 °C (scale bar, 200 nm). (g) XRD measurement of the film shown in (f). Reference lines are taken from ICDD database card 026-0575. Figure 1: CZTS nanorods and nanorod films before and after annealing. ( a ) Low resolution angular dark field transmission electron microscopy image (DFTEM) of nanorods (scale bar, 100 nm). ( b ) High-resolution transmission electron microscopy (HRTEM) image of a single rod (scale bar, 5 nm). ( c ) Top-down low resolution transmission microscopy (LRTEM) image of a monolayer sheet of vertically assembled nanorods. Inset: top-down view of a single nanorod by HRTEM (scale bar, 20 nm). The sidewalls of a nanorod are formed by lattice planes of the {100} family of the hexagonal lattice. ( d ) Cross-sectional scanning electron microscopy (SEM) image of a nanorod film (scale bar, 200 nm). ( e ) Diffractograms, measured by XRD under symmetric configuration, of two nanorod films with a high (red line) and a low (black line) degree of vertical alignment. Reference lines presenting random orientation are taken from Lu et al. [26] The nanorod drawings indicate the orientation of the nanorods within the film that contribute to the corresponding reflexes. ( f ) SEM image of a cross-section of a nanorod film after annealing at 400 °C (scale bar, 200 nm). ( g ) XRD measurement of the film shown in ( f ). Reference lines are taken from ICDD database card 026-0575. Full size image The diffractogram presented by the red line in Fig. 1e shows high intensity of the wurtzite 002 reflex compared with the vertical reference lines presenting random orientation. Since the nanorods feature elongation in c-axis direction of the hexagonal lattice, this shows that the majority of nanorods are vertically aligned with respect to the substrate surface. In contrast, the diffractogram presented by the black line shows a lower intensity of the 002 reflex, revealing that here a smaller fraction of the nanorods are vertically aligned. The inset of Fig. 1d shows that even nanorods that are not vertically oriented posses locally parallel alignment. Transition of wurtzite nanorods to large-grained kesterite To transfer wurtzite nanorod films similar to the one in Fig. 1d into kesterite CZTS films, they were annealed in an inert atmosphere on a hot plate at 400 °C (see Methods). A cross-sectional scanning electron microscopy (SEM) image of a resulting film shows that the nanorod morphology disappeared and large grains in the order of 100–300 nm formed ( Fig. 1f ). XRD reveals that the hexagonal wurtzite structure completely disappeared and tetragonal kesterite CZTS formed ( Fig. 1g ) (see Supplementary Fig. 1b for a larger angle range). Notably, all kesterite reflexes show decreased widths compared with the wurtzite reflexes of the nanorod film, which is in accordance with the increase of crystallite size [32] . The wurtzite nanorods used for this study had a Cu-poor and Zn-rich composition, which has led to the highest solar cell power conversion efficiencies in the past [8] , [11] . To study the influence of the composition on the grain growth, also nanorods with Cu-rich composition were synthesized and a similar annealing study was performed. Films made of these nanorods also showed the phase transformation to kesterite and a similar morphology after annealing ( Supplementary Fig. 2 ). It is important to note that for the formation of large grains careful washing of the nanorods for ligand removal (see Methods) is a prerequisite. When excess carbon is present in the film, only very small grain sizes are found after annealing ( Supplementary Fig. 3 ). Real-time analysis of phase transition and grain growth The correlation between phase transition and grain growth during annealing was studied in real time by synchrotron-based energy-dispersive (ED) XRD (see Methods for details). EDXRD intensities recorded every 3 s during rapid heating of a nanorod film to 500 °C are colour coded as function of time and energy in Fig. 2b . The most striking feature seen in Fig. 2a,b is a fast and direct transition from wurtzite (W) to the kesterite (K) within a few seconds at around 380±20 °C film temperature. (See Supplementary Fig. 4 for the full range of recorded data.) 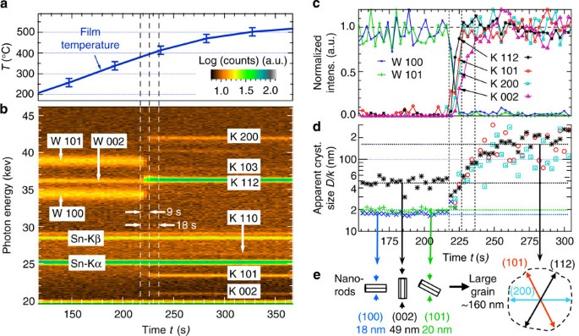Figure 2: Real-time energy-dispersive X-ray diffraction analysis during annealing of a wurtzite CZTS nanorod film. (a) Temperature of the film during annealing with a nominal maximum heating rate of 1.7 K s−1. The film temperature was determined by the thermal lattice expansion calibrated by a separate slow heating process (see Methods: Temperature estimation andSupplementary Fig. 5). (b) Colour-coded diffraction and fluorescence signals as function of photon energy and annealing time (W: wurtzite CZTS; K: kesterite CZTS; Sn-Kα and Sn-Kβ: fluorescence of Sn). To be able to resolve all wurtzite reflexes in real time, a nanorod film with a large fraction of non-vertically oriented nanorods was chosen. (c) Integral normalized intensities of kesterite (K) and wurtzite (W) reflexes obtained by multi-peak fitting. The fluctuations of the intensities before and after phase transition reflect the uncertainty of the intensities caused by limited counting statistics. (d) Apparent crystallite sizes calculated from the broadening of the diffraction signals. (e) Schematic visualization of the orientation of the different domain size dimensions as derived from (d). Figure 2: Real-time energy-dispersive X-ray diffraction analysis during annealing of a wurtzite CZTS nanorod film. ( a ) Temperature of the film during annealing with a nominal maximum heating rate of 1.7 K s −1 . The film temperature was determined by the thermal lattice expansion calibrated by a separate slow heating process (see Methods: Temperature estimation and Supplementary Fig. 5 ). ( b ) Colour-coded diffraction and fluorescence signals as function of photon energy and annealing time (W: wurtzite CZTS; K: kesterite CZTS; Sn-Kα and Sn-Kβ: fluorescence of Sn). To be able to resolve all wurtzite reflexes in real time, a nanorod film with a large fraction of non-vertically oriented nanorods was chosen. ( c ) Integral normalized intensities of kesterite (K) and wurtzite (W) reflexes obtained by multi-peak fitting. The fluctuations of the intensities before and after phase transition reflect the uncertainty of the intensities caused by limited counting statistics. ( d ) Apparent crystallite sizes calculated from the broadening of the diffraction signals. ( e ) Schematic visualization of the orientation of the different domain size dimensions as derived from ( d ). Full size image Figure 2c shows the evolution of wurtzite and kesterite reflex intensities gained by multi-peak fitting. The first vertical line in Fig. 2b and c marks the last point in time at which no kesterite reflexes are visible yet, whereas the second line marks the first point in time at which all wurtzite reflexes disappeared and kesterite reflexes are present. The distance of these two lines shows that the transformation from a hexagonal to a cubic or tetragonal lattice takes about 9 s. While the main reflexes attributed to tetragonal kesterite 112 and 200 could also stem from a cubic phase, the occurrence of the weak 101 and 002 reflexes reveals formation of tetragonal CZTS. The rise of the intensities of these weak reflexes relative to the intensities of the main reflexes provides valuable insight into the dynamics of cation ordering within the sulphur sublattice after transformation from the wurtzite to the tetragonal structure. Lattice defects involving Sn such as (Sn Cu +Cu Sn ) or (Sn Zn +Zn Sn ) antisite pairs may strongly affect the electronic properties such as a decreased band gap energy [33] , which might lead to detrimental band gap fluctuations. Our experiment is sensitive to Sn-Cu and Sn-Zn disorder. If Sn ions were randomly distributed over the Sn and Zn sites, the 002 reflex would be completely cancelled out (see Supplementary Fig. 6 ). If, moreover, Sn would be randomly distributed over all cation sites including the Cu sites, the 101 reflex would be cancelled out as well. Therefore, the simultaneous occurrence of the 101 reflex with the main 112 and 200 reflexes ( Fig. 2c ) reveals a fast ordering of the Cu site occupation, avoiding occupation by Sn ions. In contrast, the rise of the 002 reflex shows a small delay compared with the other signals ( Fig. 2c ). While it should be noted that this delay is small compared with the scattering of the signal intensities, a possible explanation could be an initial Sn-Zn disorder with subsequent quick decay of this disorder. The quick decay of the Sn-Zn disorder would be in accordance with a theoretically predicted high formation energy of (Sn Zn +Zn Sn ) antisite pairs [33] . We conclude that the complete kesterite formation with ordered Sn cation site occupation takes about 18 s, as marked by the third line in Fig. 2b and c . We note that the real-time data are not sensitive to Cu–Zn disorder resulting in so-called disordered kesterite [34] , [35] , [36] –which, however, is predicted to be less critical for the electronic structure of CZTS [33] , [34] . The evolution of grain growth is monitored by the broadening of the diffraction reflexes. The reflexes of the wurtzite nanorods show a strong variation in peak width for different lattice plane orientations ( Fig. 2b ). The apparent crystallite sizes calculated from the corrected integral widths of the wurtzite reflexes are consistent with the nanorod shape ( Fig. 2d,e ) (see also Methods: Calculation of crystallite size). We note that the size of the nanorods is overestimated compared with the dimensions revealed by high-resolution transmission electron microscopy ( Fig. 1b ). This can be explained by a partial coherence of the lattices of aligned nanorods [37] . Figure 2d shows that the size and shape of the wurtzite nanorods stay constant up to the point of phase transition. In contrast, the sizes of the kesterite crystals as calculated from the various diffraction signals do not show a dependence on the orientation and quickly increase until their average diameters are larger than the size of the original nanorods ( Fig. 2d,e ). This interpretation of the real-time signals is supported by cross-sectional SEM images of nanorod films heated to three different temperatures ( Fig. 3 ). 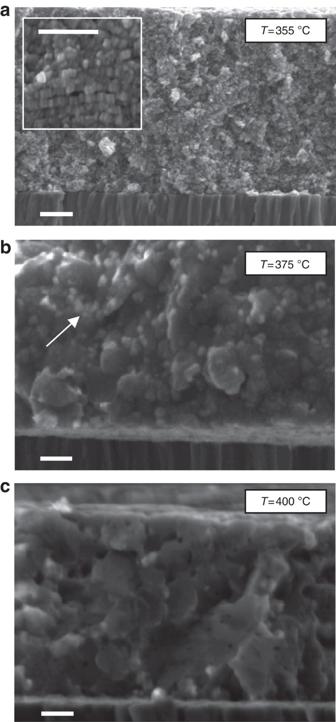Figure 3: Cross-sectional SEM images of nanorod films annealed at three different temperatures. (a) The film annealed to 355 °C still shows nanorods of original size (scale bars, 200 nm). (b) The film annealed to 375 °C already shows some larger grains, but also still some small crystallites (marked by white arrow) near the size of the original nanorods (scale bar, 200 nm). (c) Finally, the film annealed to 400 °C shows only large grains (scale bar, 200 nm). Figure 3: Cross-sectional SEM images of nanorod films annealed at three different temperatures. ( a ) The film annealed to 355 °C still shows nanorods of original size (scale bars, 200 nm). ( b ) The film annealed to 375 °C already shows some larger grains, but also still some small crystallites (marked by white arrow) near the size of the original nanorods (scale bar, 200 nm). ( c ) Finally, the film annealed to 400 °C shows only large grains (scale bar, 200 nm). Full size image Heating rate variation To investigate the influence of the heating rate on the phase transition, additional real-time measurements during annealing of a nanorod film were performed with the same conditions as for the process shown before in Fig. 2 except that the heating rate was drastically reduced from 1.7 K s −1 to 0.05 K s −1 . While for the slower heating rate the phase transition also proceeds from the wurtzite directly to the kesterite phase ( Supplementary Fig. 4 ), the phase transition is shifted to lower temperature—as is expected if the transition is thermally activated. Interestingly, however, the reduction in heating rate results in substantially broader diffraction lines of the final kesterite phase ( Fig. 4a ), indicating smaller final size of the kesterite domains and hence a strong reduction in grain growth. 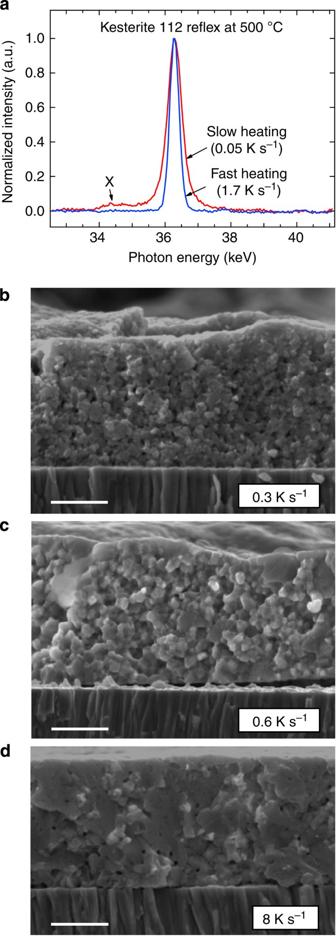Figure 4: Influence of heating rate on the microstructure. (a) Comparison of the width of the kesterite 112 reflex at 500 °C for the fast and the slow heating process. ‘X’ marks a signature that can be attributed to stacking faults in the tetragonal S sublattice38. (b–d) SEM images on cross-sections of nanorod films after heating to 500°C, showing increasing grain size with increasing heating rate (scale bars, 500 nm). No obvious further increase in grain size with heating rate could be observed above 2.6 K s−1, which shows similar morphology as 8 K s−1. Figure 4: Influence of heating rate on the microstructure. ( a ) Comparison of the width of the kesterite 112 reflex at 500 °C for the fast and the slow heating process. ‘X’ marks a signature that can be attributed to stacking faults in the tetragonal S sublattice [38] . ( b – d ) SEM images on cross-sections of nanorod films after heating to 500 ° C, showing increasing grain size with increasing heating rate (scale bars, 500 nm). No obvious further increase in grain size with heating rate could be observed above 2.6 K s −1 , which shows similar morphology as 8 K s −1 . Full size image The signature on the left-hand side in Fig. 4a marked with ‘X’ can be attributed to planar faults in the 112 planes of the tetragonal S sublattice [38] , causing hexagonal subdomains, which might be inherited from the original wurtzite structure. This signature makes reliable analysis of the crystallite sizes for the slow heating process from the diffraction data difficult. Therefore, the morphology of films annealed with various heating rates was analysed ex situ by cross-sectional SEM. Figure 4b–d clearly show that the grain size significantly increases with increasing heating rate. Electrical and optical characterization From the large microstructural differences imposed by the heating rate variation, the question arises how these differences affect the semiconductor properties of the film. To answer this question, we performed electrical and optical characterization of the CZTS nanorod films before and after annealing with various heating rates. Electrical transport properties were characterized by a four probe measurement set-up (see Methods for details). For sample preparation, CZTS nanorod solution was spin-coated onto glass substrates to get nanorod films with uniform thickness. For the as-deposited nanorod films the conductivity is below the detection limit of the instrument. This can be expected due to long chain non-conductive ligand shell on the nanorod surface and nanometre sized gaps between the single rods ( Fig. 1c ). Subsequently, nanorod films were heated to 500 °C. When heating with a slow heating rate (0.3 K s −1 ), which leads to formation of small grains ( Fig. 4 ), the films show an average conductivity of 4.1 × 10 −3 Ω −1 cm −1 (average from six samples). When heating with a fast heating rate (above 2.6 K s −1 ), which leads to formation of larger grains, the films show increased conductivity, with an average of 2.5 × 10 −2 Ω −1 cm −1 (average from 14 samples). This value is comparable with conductivities observed for CZTS films prepared by sulfurization of metallic precursors [39] , which is an approved method for fabrication of CZTS solar cells [40] , [41] , [42] . Above a heating rate of 2.6 K s −1 no systematic dependency on the heating rate could be observed. While the measured values obtained for the fast heating rates are quite disperse and range from 1.5–4.9 × 10 −2 Ω −1 cm −1 , these values all lie above those from the slowly heated samples, ranging from 2.6–7.4 × 10 −3 Ω −1 cm −1 . While the electrical conductivity might be influenced by many factors, the lower conductivity of the slowly heated samples could be explained by a higher density of grain boundaries, which might form barriers for the charge carriers. Further, Raman analysis was performed to investigate phase purity and crystal quality of the annealed films as a function of the heating rate. The Raman spectra of a CZTS wurtzite nanorod film as well as samples heated with several heating rates are presented in Fig. 5a . The observed Raman peaks at 150, 260, 288, 338 (A-mode), 366 and 376 cm −1 (vertical lines in Fig. 5a ) are in good agreement with peak positions earlier found for kesterite CZTS [43] , while dominant modes at 334 and 377 cm −1 (arrows) of CZTS nanorods have been also reported for wurtzite CZTS [10] , [20] . The strongest A-mode symmetry of kesterite CZTS of the annealed samples shifts to lower frequencies and significantly broadens with decreasing heating rate as shown in the inset of Fig. 5a . This shift of the A-mode can be explained by an increase in disorder in the kesterite cation sublattice [44] as well as possible remnants of the wurtzite-type structure. The latter matches with the observation of an additional diffraction signal in slowly heated films ( Fig. 4a , signal ‘X’), which was attributed to the presence of hexagonal type planar faults (such as stacking faults) within the kesterite phase, possibly inherited from the original wurtzite nanorods. Thus, the Raman results in Fig. 5a indicate improving structural quality of the CZTS films with increasing heating rate. 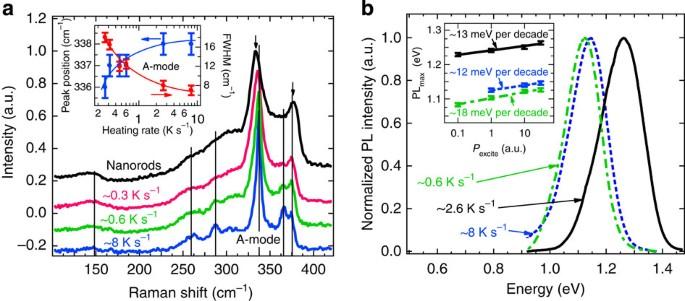Figure 5: Influence of heating rate on film properties. (a) Raman spectra for the as-deposited CZTS nanorod precursor film and for annealed samples heated with three different heating rates 0.3, 0.6 and 8 K s−1. The signals of the annealed films at 150, 260, 288, 338 (A-mode), 366 and 376 cm−1(vertical lines) can be attributed to kesterite43. The arrows at 334 and 377 cm−1mark the positions of the wurtzite signals10,20. The inset shows peak position and full width at half maximum (FWHM) of the main kesterite peak (A-mode) as function of heating rate. The lines are guides to the eye. (b) Low temperature photoluminescence (PL) intensities measured at 10 K for annealed films heated with three different heating rates. The inset shows PL peak positions (PLmax) as function of excitation power (Pexcite). Figure 5: Influence of heating rate on film properties. ( a ) Raman spectra for the as-deposited CZTS nanorod precursor film and for annealed samples heated with three different heating rates 0.3, 0.6 and 8 K s −1 . The signals of the annealed films at 150, 260, 288, 338 (A-mode), 366 and 376 cm −1 (vertical lines) can be attributed to kesterite [43] . The arrows at 334 and 377 cm −1 mark the positions of the wurtzite signals [10] , [20] . The inset shows peak position and full width at half maximum (FWHM) of the main kesterite peak (A-mode) as function of heating rate. The lines are guides to the eye. ( b ) Low temperature photoluminescence (PL) intensities measured at 10 K for annealed films heated with three different heating rates. The inset shows PL peak positions (PL max ) as function of excitation power ( P excite ). Full size image As photoluminescence (PL) probes radiative recombination paths of charge carriers, it provides essential information on the quality of semiconductor materials and their suitability for photoelectrical devices. Low-temperature PL spectra of some CZTS annealed samples are displayed in Fig. 5b . The emission is dominated by a broad band centred in the range from 1.1–1.3 eV with full width at half maximum of about 0.2 eV. The PL peak position blue shifts by 10–20 meV per decade with increasing excitation power (inset of Fig. 5b ), indicating strong compensation, which has been found to be a necessary prerequisite for good solar cell performance in chalcopyrite as well as kesterite-based thin film solar cells [45] , [46] , [47] . The observed PL bands in CZTS annealed samples can be attributed to quasi donor–acceptor recombination [45] , [46] . We do not find an obvious trend for the influence of the heating rate on the PL properties of the annealed CZTS films. This finding implies that the radiative recombination paths in the CZTS films are not predominantly affected by differences in the microstructure induced by the heating rate variations. The real-time data presented in Fig. 2 revealed a direct correlation between phase transition and grain growth during fast heating. It was shown that a reduction in the heating rate leads to a strong reduction of grain growth ( Fig. 4 ). Without any grain growth, each wurtzite nanorod could be expected to transform individually to kesterite. Such a transformation corresponds to a simple first-order reaction where the reaction rate is proportional to the concentration of the reactant c W : −d c W /d t =+d c K /d t = c W ( t ) A exp[− E a / k B T ( t )] ( c W and c K are the concentrations of wurtzite and kesterite expressed as molar fraction, t is the time, A a pre-exponential factor, E a the thermal activation energy, k B the Boltzmann constant and T the temperature). Integration with respect to time yields (see Method: First-order reaction). The dashed and solid orange lines in Fig. 6a show that this equation describes the phase transition measured during slow heating very well. In contrast, the fast heating process shows a strong deviation between the intensities of the measured kesterite signals ( Fig. 6b , black circles) and the intensities corresponding to the first-order reaction calculated with the same parameters as for the slow heating ( Fig. 6b , orange line): whereas the first-order reaction correctly describes the onset of the measured kesterite formation, the subsequent increase of the measured signals is much steeper. This steep increase of the kesterite signals and the simultaneous onset of grain growth ( Fig. 6c ) suggest that the phase transition is enhanced by growth of kesterite grains, while grain growth itself is triggered by the transition from the wurtzite to the kesterite phase. 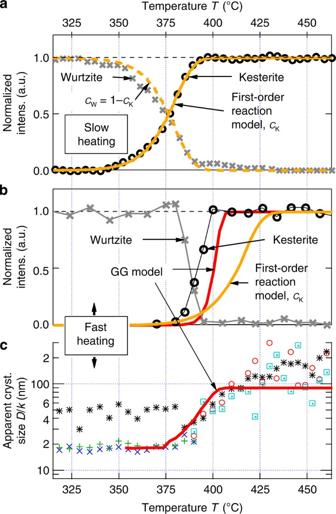Figure 6: Comparison of the numerical modelling with the experimental data. (a,b) Evolution of the phase transition as function of temperature during (a) slow heating with a heating rate of 0.05 K s−1and (b) fast heating with a heating rate of 1.7 K s−1. The crosses and circles mark measured, normalized wurtzite and kesterite diffraction intensities. For the fast heating, several representative intensities were averaged in order to reduce noise. The orange lines correspond to the first-order reaction model of Equation (1) withEa=3.54 eV andA=1.1 × 1025s−1. (c) Evolution of the crystallite size as calculated from the EDXRD signal broadening during fast heating. The red lines in (b) and (c) correspond to the phase-transition-driven grain growth model (GG model). Figure 6: Comparison of the numerical modelling with the experimental data. ( a , b ) Evolution of the phase transition as function of temperature during ( a ) slow heating with a heating rate of 0.05 K s −1 and ( b ) fast heating with a heating rate of 1.7 K s −1 . The crosses and circles mark measured, normalized wurtzite and kesterite diffraction intensities. For the fast heating, several representative intensities were averaged in order to reduce noise. The orange lines correspond to the first-order reaction model of Equation (1) with E a =3.54 eV and A =1.1 × 10 25 s −1 . ( c ) Evolution of the crystallite size as calculated from the EDXRD signal broadening during fast heating. The red lines in ( b ) and ( c ) correspond to the phase-transition-driven grain growth model (GG model). Full size image To understand this behaviour, we take a closer look at the structural differences of the wurtzite and kesterite phases. In the wurtzite nanorods, the sidewalls are formed by {100} planes ( Fig. 1c ) and hence surface atoms have three bonds ( Fig. 7a ). As no surface with more bonds per atom exists, the sidewalls can be expected to be relatively stable compared with other planes. A phase transition from the hexagonal wurtzite to the tetragonal kesterite phase can be seen as a shift of every third layer of sulphur atoms ( Fig. 7a,b ). Starting from the original nanorod shape, this would result in sidewall atoms that only have two bonds ( Fig. 7b ). However, kesterite surfaces formed by {112} planes, in which every atom has three bonds, are energetically preferred [48] . Hence, it can be assumed that the shape of the nanorods is not preserved during phase transition, which unavoidably brings the boundary of the newly formed crystal (seed crystal) closer to the neighbouring nanorods ( Fig. 7c ). We propose that this stimulates the transition of the metastable wurtzite lattice of the neighbouring nanorods to the kesterite lattice of the seed crystal, thereby causing the seed crystal to grow. As a crystal grows, it comes into contact with more and more nanorods ( Fig. 7d ). Consequently, the rate of volume growth can be expected to be proportional to its surface, which corresponds to normal grain growth [49] . According to this model, the transition from nanorods to larger grains and the phase transition from wurtzite to kesterite occur simultaneously, which is in agreement with the real-time analysis ( Fig. 2 ). 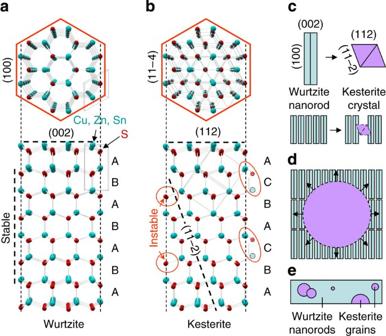Figure 7: Consequences of the structural differences between wurtzite and kesterite for the transition from wurtzite nanorods to kesterite grains. (a) Structure of a wurtzite nanorod. For simplicity, the number of atoms is reduced. (b) Structure of a kesterite or sphalerite crystal with a shape close to the nanorod shape. (c–e) Illustration of the model of phase-transition-driven growth of kesterite grains within a template of metastable wurtzite nanorods. Figure 7: Consequences of the structural differences between wurtzite and kesterite for the transition from wurtzite nanorods to kesterite grains. ( a ) Structure of a wurtzite nanorod. For simplicity, the number of atoms is reduced. ( b ) Structure of a kesterite or sphalerite crystal with a shape close to the nanorod shape. ( c – e ) Illustration of the model of phase-transition-driven growth of kesterite grains within a template of metastable wurtzite nanorods. Full size image The main steps of this reaction are (1) the transition from a wurtzite to a kesterite nanocrystal (nucleation) and (2) the growth of this crystal by incorporation of further nanocrystals (grain growth). According to this picture, the final average grain size will depend on the relation between the nucleation rate and the growth rate, and hence on the difference of the activation energies for nucleation ( E N ) and growth ( E G ). If E N < E G , and if the heating rate is sufficiently slow, all nanorods will individually transform to kesterite crystals before the mechanism for grain growth becomes active, resulting in a small final grain size. In contrast, at higher heating rates the reaction is shifted to higher temperatures ( Fig. 6a,b ) and hence the grain growth can become active during the phase transition, resulting in larger final grain sizes, which qualitatively matches our findings ( Fig. 4 ). To test if this model can describe the experimental observed correlation of grain growth and phase transition, we performed numerical three-dimensional model calculations: the thermally activated transformation of single nanorods to kesterite seed crystals is realized by a simple Monte-Carlo procedure, where the probability for the transformation of a nanorod is given by an Arrhenius equation with activation energy E N =3.5 eV. Subsequent growth is described by a second Arrhenius equation determining the increase per time step of the radius of a spherical grain with activation energy E G =3.8 eV. This procedure leads to the coexistence of grains with different sizes ( Fig. 7e ). The model takes into account that via this phase-transition-driven grain growth, kesterite grains can only grow where their surface is in contact with wurtzite nanorods. Hence, they stop to grow where they come into direct neighbourhood with other kesterite grains ( Fig. 7e ). (For further details see Methods: Modelling.) The evolution of the integral molar fraction of the kesterite phase as well as the volume weighted grain size resulting from this grain growth (GG) model calculation are added as red lines to Fig. 6b and c . The comparison with the experimental data confirms that the proposed model describes well the tendency of the observed correlation between phase transition and grain growth. We conclude that growth of kesterite grains within a template of ordered wurtzite nanorods is driven by the transition from the metastable to the stable crystalline phase. Via this reaction, large-grained tetragonal Cu 2 ZnSnS 4 films can be formed within a few seconds. The number of grains and their average grain size can be controlled by the heating rate, where fast heating leads to larger grains. By designing size and arrangements of precursor nanorod clusters, this reaction route could be utilized to synthesize semiconductor crystals for nano- and microstructured photoelectric devices. Chemicals Copper(II) acetylacetonate (Cu(acac)2, >99.99%), Tin(IV) acetate (Sn(OAc)4, >99.99%), Zinc acetate (Zn(OAc)2, >99.99%), trioctylphosphine oxide (TOPO, 99%), 1-octadecene (ODE, 90% tech), 1-dodecanethiol (1-DDT, 98%), tert-dodecylmercaptan (t-DDT), Oleylamine (technical grade, 70%) were purchased from Aldrich. All chemicals were used as received without any further purification. Synthesis of wurtzite CZTS nanorods Cu 2 ZnSnS 4 (CZTS) nanorods were synthesized by using a modification of our previously published procedure [20] . Cu(acac)2 (1.332 mmol), Zinc acetate (0.915 mmol), Tin(IV) acetate (0.75 mmol) and TOPO (4 mmol) were mixed with 10 ml of ODE in a 25 ml three-neck flask and evacuated at room temperature for 30–45 min. The solution was then heated to 250–270 °C in 15–20 min under an argon atmosphere, and at 155 °C, a mixture of 0.5 ml 1-DDT and 3.5 ml t-DDT was injected into the flask. This resulted in an immediate colour change from dark green to wine-red and then finally to brown. After injection, the reaction was allowed to proceed for 30 min with continuous stirring. Subsequently, the heating mantle was removed and the reaction vessel was allowed to cool to 80 °C. 2–3 ml of anhydrous toluene was added swiftly to quench the reaction. The nanorods were then washed 2–3 times in a 2:1 ratio of toluene to ethanol (anhydrous) and centrifuged at 4,000 r.p.m. for 10 min to yield a dark brown centrifuged product. The nanorods are re-dispersed in anhydrous toluene and stored in a glove box for the further experiment. The as-synthesized nanorod has a Cu/(Zn+Sn) ratio of 0.8 and a Zn/Sn ratio of 1.2, which is close to thin film photovoltaic devices with highest reported power conversion efficiencies [8] , [11] . For the copper-rich nanorod sample (Cu/(Zn+Sn)=1.05 and Zn/Sn=1), copper(II) acetylacetonate (1.05 mmol), Zinc acetate (0.5 mmol), Tin(IV) acetate (0.5 mmol), TOPO (3.5 mmol), 10 ml of ODE and thiols mixture (0.25 ml 1-DDT and 1.75 ml t-DDT) were used. Other reaction and washing conditions were similar as for copper poor nanorod synthesis. Electrophoretic deposition A custom-made gold-coated copper electrode (parallel) with a separation of 5 mm apart was used for nanorod deposition. A toluene solution of CZTS nanorods (20–25% w/v) was used for electrophoresis. Before deposition, the nanorod solution is sonicated for 10–15 min to get well dispersion of nanorods in toluene. During electrophoresis, the Mo-coated soda lime glass substrates (12 mm × 15 mm) were attached onto the negative electrodes. The electrodes were completely immersed in a nanorod solution and a potential of 300–500 V was applied to the substrate for 3–5 min using a high voltage power supply unit (TECHNIX SR-5-F-300, S/N: BU08/04971) and voltage was monitored using Black star 3225 MP millimetre. After deposition, the electrodes are pulled out from nanorod solution bath and dried slowly under solvent saturation environment. The Mo-glass substrate is put in the desiccator to remove all solvent before further characterization. Ex-situ annealing experiment set-up For ex-situ annealing experiments, CZTS nanorod films on Mo-substrate are annealed on a hot plate at different temperatures of 355, 375, 400 and 500 °C in an argon glove box for 10–15 min. For the heating rate variations, all samples were heated up to 500 °C and held at 500 °C for 10 min. After annealing, the substrate is allowed to cool down to room temperature and cleaved for cross-sectional SEM analysis. In-situ annealing experiment set-up For the real-time EDXRD analysis, nanorod films were annealed in a sealed reaction box inside a vacuum chamber coupled to the polychromatic synchrotron beamline EDDI at BESSY II [50] . EDXRD is particularly suitable for highly time-resolved observations of kesterite formation since the diffraction angle can be adjusted such that the energy positions of the low intensity kesterite reflexes 101, 110 and 002—which are important for the discrimination of kesterite from the structurally related secondary phases such as Cu 2− x Se, ZnS and Cu 2 SnS 3 —coincide with the energy range with highest photon flux [51] of the polychromatic synchrotron beam. In addition, changes in domain sizes of crystalline material can be monitored in real-time via the broadening of diffraction lines as a function of time [52] . The films were heated to 500 °C with a nominal heating rate of 1.7 or 0.05 K s −1 by the radiation of eight halogen lamps with a total power of 4 kW. The temperature was controlled with a thermocouple positioned above the film. Before annealing, the reaction box was evacuated until a pressure of 10 −4 mbar was reached. Subsequently, the reaction box was sealed by a motor valve. The reaction box consists of a pyrolytically coated graphite cylinder, which is closed by quartz plates at the bottom and top. More details on the set-up can be found in (ref. 53 ). The annealing chamber is equipped with two polyimide windows for synchrotron radiation. During the processes, diffraction and fluorescence signals were recorded with an energy-dispersive high-purity Ge detector and a scattering angle of 2 θ =6.24°. The relationship between lattice plane distance d hkl of a crystalline phase and the photon energy E hkl of the corresponding diffraction line follows the energy-dispersive Bragg law E hkl = hc /(2 d hkl sin( θ )), where h is Planck’s constant, and c the speed of light. EDXRD data analysis Integral intensities and integral widths of the EDXRD reflexes were gained by fitting the signals with Voigt profiles using the software package IGOR Pro 6. Owing to a similar position of the wurtzite 002 and kesterite 112 reflexes ( Fig. 2 )—which reflects the close structural relationship and similar density of these phases—they cannot be separated and thus were fitted with a single Voigt profile. The normalized intensity increase of this signal was attributed to an increase of the kesterite 112 reflex. Temperature estimation: During the heating ramp (1.7 K s −1 ) of the fast heating process shown in Supplementary Fig. 4 (left), the temperature measured by the thermocouple placed above the sample may deviate from the film temperature due to differences in the thermal mass and absorption coefficient of thermocouple and sample. During the slow heating with a heating rate of 0.05 K s −1 , it can be assumed that the temperature of the thermocouple is much closer to that of the film, because the mentioned differences play a smaller role. Here, the accuracy of the temperature measurement is assumed to be ±20 K. We use the thermal expansion of the wurtzite and the kesterite phase measured during slow and fast heating to estimate the true temperature of the film during fast heating. Supplementary Fig. 5a and b show the lattice plane spacings for the wurtzite (W) and kesterite (K) phase during slow heating. The data were fitted with a straight line. From this, the following linear thermal expansion coefficients are derived: CZTS-W (100): α =(4.83 × 10 −6 ±0.09 × 10 −6 ) nm K −1 CZTS-W (101): α =(4.14 × 10 −6 ±0.06 × 10 −6 ) nm K −1 CZTS-K (101): α =(6.14 × 10 −6 ±0.19 × 10 −6 ) nm K −1 . Supplementary Fig. 5d and e show the values of the lattice plane spacings measured during the fast heating process. With the help of the thermal expansion coefficients given above, the temperature was calculated from these lattice plane spacings. The temperatures resulting from this calculation are given in Supplementary Fig. 5f as dots. The dashed black line results from concatenating and smoothing of the calculated temperatures. The arrow bars reflect the uncertainty of the temperature measurement of ±20 K during the slow heating. For comparison, the calculation of the temperature out of the measured lattice plane spacings and the expansion coefficients was also done for the slow heating process, as shown in Supplementary Fig. 5c . Calculation of crystallite size The apparent crystallite sizes were calculated from the integral width β f of the physical diffraction line profiles of each recorded EDXRD spectrum (the term crystallite is understood as domain of undisturbed coherent scattering). To obtain β f , the measured profiles were fitted by a Voigt profile V h ( E ) using the parameterization of Humlicek [54] implemented in the software package IGOR Pro 6. The Gaussian contribution β h,G to the width of V h ( E ) was corrected by the Gaussian shaped broadening β g,G caused by the experimental set-up: β f,G =( β h,G 2 – β g,G 2 ) 1/2 . Since the experimental set-up causes a purely Gaussian shaped broadening, the Lorentz contribution to the width of the physical Voigt profile β f,L equals that of the measured profile: β f,L = β h,L . The total integral width of the physical Voigt profile β f was calculated from the Gauss and the Lorentz width β f,G and β f,L with the help of the parameterization of Humlicek [54] . The calculation of the apparent crystallite sizes follows the energy-dispersive form of Scherrer’s equation [55] D / k = hc /(2 β f ·sin( θ )) (with θ= 3.12°), and assumes that the measured profiles are only broadened by the crystallite sizes and by the resolution of the experimental set-up. For the CZTS nanorods, this assumption is justified by the undisturbed crystal structure revealed by high-resolution transmission electron microscopy ( Fig. 1b of the main text). Electrical and optical characterization Electrical transport properties were characterized by using a four probe measurement set-up inside the glove box. The measurements were performed with a 2400 source meter from Keithley Instruments and the conductivity of the thin films was measured under dark condition at ambient temperature. Four ohmic contacts (gold) were deposited on the corner of the substrates by thermal evaporation to avoid electrical contact problems on the film. The conductivity was measured by the van der Pauw method. Room temperature Raman spectra were measured in the back-scattering configuration using a He−Ne (wavelength 632.8 nm) laser in a DILOR LabRam Micro-Raman system. The CCD detection system was calibrated with respect to 520.7 cm −1 peak position of a reference silicon wafer. Low-temperature PL measurements were performed at 10 K using a 660 nm laser diode and 0.25 m grating monochromator equipped with an InGaAs detector array with the samples mounted in a closed-cycle He cryostat. First-order reaction From the real-time diffraction data recorded during slow heating we follow that the reaction implies a direct transition from the reactant (wurtzite CZTS) to the product (kesterite CZTS). This means that the reaction rate r can be assumed to be proportional to the concentration c W of the reactant (wurtzite CZTS) and that the concentration of the product (kesterite CZTS) is c K =1– c W , if the concentrations are expressed as molar fractions. Further, we assume that the reaction is thermally activated. Such a reaction is described by the Arrhenius equation of first order: where r is the reaction rate, A is a constant factor, E a the activation energy, k B the Boltzmann constant and T the temperature of the sample. Since in our experiment the temperature continuously changes as a function of time t , we replace T by T ( t ) and integrate over time: c W,0 is the initial molar fraction of wurtzite CZTS and was set to 1. The integration was solved numerically. A least square fit using the Levenberg–Marquardt algorithm of the software IGOR Pro 6 was performed to determine the parameters A and E a for which the function c K ( t ) best matches the evolution of the normalized intensity of the K 112 signal ( Fig. 6a ). As this signal overlaps with W 002, for the normalization the initial intensity was subtracted from all intensity values and then the intensity values were divided by the final intensity. This normalized intensity is taken as representative of the concentration of kesterite CZTS. The least square fit gave the following fit parameters: E a =(3.54±0.03) eV; A =(1.1±0.7)·10 25 s −1 . The given errors result from the accuracy of the fit and do not account for the uncertainty of the measured temperature. An addition of 20 K to the temperature profile yields: E a =(3.77±0.04) eV; A =(9±6)·10 25 s −1 A subtraction of 20 K to the temperature profile yields: E a =(3.34±0.03) eV; A =(0.21±0.13)·10 25 s −1 . We use the difference of the resulting activation energies for the estimation of its error limit: E a =(3.5±0.3) eV. Modelling of phase-transition-driven grain growth We implemented a numerical code to calculate the evolution of phase transition expected from the model of phase-transition-driven grain growth. In this model, the formation of kesterite seed grains is thermally activated and its probability within a given time step at a given temperature is described by an Arrhenius equation. The nucleation rate is proportional to the remaining reactant, that is, to the unreacted wurtzite nanorods. In addition, the grain growth is assumed to be proportional to the grains surface and determined by a second Arrhenius equation. This means that at constant temperature, the radius of the grains would increase linearly with time, which corresponds to normal grain growth. The shape of the grains is approximated by spheres. At parts of a grains surface at which it is in direct neighbourhood with other grains or with the film surface, it does not further grow. Consequently, in this model the growth stops when all wurtzite transformed into kesterite. According to this model, the phase transformation consists of two steps. First, the transformation of a single wurtzite nanorod to a kesterite grain (see Nucleation). Second, the growth of the kesterite grain by incorporation of material of wurtzite nanorods at the grain surface (see Grain growth). The time and temperature dependent progress of nucleation and grain growth are numerically modelled by means of a time discretization, where both mechanisms are sequentially treated at each time step. Nucleation For the nucleation, the number of newly created kesterite seed grains (Δ N K ) in a time interval Δ t is calculated by the following equation: where N W is the total number of remaining wurtzite crystals, A N is the pre-exponential factor, E N is the activation energy for the nucleation, k B is the Boltzmann constant and T ( t ) is the temperature as function of time. In general the equation gives a rational number. This number is taken as probability and the number of actually newly created kesterite grains (Δ N K,act ) is determined by using a random number generator such that floor (Δ N K )<Δ N K,act < ceil (Δ N K ) and ‹ΔN K,act ›=ΔN K (where the operation ‘floor’ rounds down and the operation ‘ceil’ rounds up to the next integer). The brackets in ‹ Δ N K,act ›=Δ N K say that the average number of actually created seeds will equal to Δ N K if this operation is repeated infinitely often. Another random number generation is deployed to randomly choose the location of the newly created seed grains, taking into account that this can only happen where wurtzite has not already transformed into kesterite. We note that without additional grain growth the evolution of phase transition obtained by this procedure coincides with the first-order reaction described by equation (1) of the main text. To be able to distinguish between different grains, each grain is given a unique identification number (ID) when it is created. For each grain, the time at which it was created (nucleation time t N ) is recorded. This information is needed for the calculation of the grain growth. Grain growth Once a grain is created, its new size characterized by its radius is determined after each time interval. The radius at time t of a single grain created at nucleation time t N with an initial radius R N is calculated by where A G is the pre-exponential factor and E G the activation energy for grain growth. The integral was solved numerically. For each grain, each volume unit lying inside the increased volume of the grain is attributed to this grain if the volume unit was not attributed to a different grain before. Each volume unit that is attributed to a grain is marked by the ID of the grain. Determination of phase transition The evolution of phase transition is obtained at each time interval by counting the volume units that are attributed to any of the kesterite grains. This value is normalized to the total sample volume used for the modelling. Consequently, complete phase transition is reached if this normalized value reaches unity. Determination of volume weighted grain size Signal broadening of XRD is sensitive to the volume weighted length of undisturbed crystal structure perpendicular to the scattering lattice plane, that is—in a symmetric diffraction set-up—perpendicular to the sample surface. Therefore, the average volume weighted size of all kesterite grains was determined by counting the length of each vertical array of volume units possessing equal grain ID’s. This procedure assumes that a grain consists of a single domain of coherent scattering. Modelling parameters The maximum number of possible nucleation sites was 250,000, and R N was set to 10 nm. The sample volume was set to 2.5 × 10 8 nm 3 . T ( t ) was taken from the estimated temperature profile shown in the left of Supplementary Fig. 4 . Δ t was 1 s, and the Arrhenius parameters used for the nucleation and grain growth were E N =3.5 eV, A N =4 × 10 22 s −1 , and E G =3.8 eV, A G =3 × 10 29 s −1 . How to cite this article : Mainz, R. et al. Phase-transition-driven growth of compound semiconductor crystals from ordered metastable nanorods. Nat. Commun. 5:3133 doi: 10.1038/ncomms4133 (2014).